Arene dearomatization through a catalytic N-centered radical cascade reaction Arene dearomatization reactions are an important class of synthetic technologies for the rapid assembly of unique chemical architectures. Herein, we report a catalytic protocol to initiate a carboamination/dearomatization cascade that proceeds through transient sulfonamidyl radical intermediates formed from native sulfonamide N–H bonds leading to 1,4-cyclohexadiene-fused sultams. Importantly, this work demonstrates a facile approach to employ two-dimensional aromatic compounds as modular building blocks to generate richly substituted, three-dimensional compounds. These reactions occur at room temperature under visible light irradiation and are catalyzed by the combination of an iridium(III) photocatalyst and a dialkyl phosphate base. Reaction optimization, substrate scope, mechanistic features, and synthetic applications of this transformation are presented. Arenes obtained from inexpensive petrochemical feedstocks are incorporated on industrial scale into pharmaceuticals, agrochemicals, and organic materials. Selective dearomatization reactions [1] , [2] of these flat, two-dimensional aromatic compounds are modular strategies to access substituted, three-dimensional chemical space [3] , including fused, complex heterocyclic skeletons [4] , [5] . In addition, the potential to form stereogenic centers through substituent addition concomitant with the dearomatization process is particularly appealing. Of the selective dearomatization methods reported (including UV-promoted photochemical cycloadditions [6] , [7] , oxidative [8] , enzymatic [9] , [10] , [11] , transition metal-mediated [12] , [13] , [14] , and nucleophilic dearomatizations [15] ), the Birch reduction of arenes to 1,4-cyclohexadienes (1,4-CHD) is most well-known relying on liquid ammonia as solvent and pyrophoric alkali metals at cryogenic temperatures (Fig. 1a ) [16] , [17] . Modifications of the canonical Birch reduction conditions have expanded the scope and synthetic utility of the reaction [18] , [19] , [20] , [21] , [22] . Although both electrochemical [23] and visible light-mediated [24] , [25] , [26] , [27] , [28] arene dearomatization reactions have been reported with proven utility, they have not been integrated with other reaction pathways via reactive intermediates. A complementary strategy addressing the inherent drawbacks of the classic Birch reduction is to promote an arene dearomatization via a radical cascade sequence. Radical cascades, processes in which multiple chemical bonds are formed in a single operation, are step and atom-economical means to rapidly build complex organic molecules (Fig. 1b ) [29] , [30] , [31] . Moreover, initiating cascade sequences from strong N–H bonds leading to dearomatized molecular frameworks has the potential to impact a variety of synthetic endeavors. Fig. 1: Inspiration and design for our carboamination/dearomatization cascade reaction platform. a The classic Birch reduction for arene dearomatization. b The design principle of using a radical cascade approach for arene dearomatization. c This work: catalytic radical carboamination/dearomatization cascade reactions. Full size image Multiple-site concerted proton-electron transfer (MS-CPET) has emerged as a powerful strategy for homolytic activation of strong N–H bonds, often in the presence of weaker ones, avoiding the need for N -pre-functionalization [32] , [33] , [34] . The Knowles group recently reported the activation of both amide [35] and sulfonamide [36] N–H bonds for intramolecular and intermolecular hydroamination reactions, respectively, of electron-neutral olefins. The authors propose an excited-state redox catalyst and a weakly coordinating phosphate base, jointly mediate the concerted homolytic activation of the strong N–H bonds under visible light irradiation to afford transient N -centered amidyl and sulfonamidyl radicals capable of adding to olefins with anti -Markovnikov regioselectivity. Separately, Chu and Rovis [37] described the generation of amidyl radicals from trifluoroacetamide derivatives for sequential 1,5-HAT and δ-C–H functionalization. By using superstoichiometric K 3 PO 4 as the base, trifluoroacetamides are deprotonated to the amidyl anions then oxidized to the amidyl radical by the excited state of an iridium(III) photocatalyst. With respect to sulfonamide-based N -radical alkene carboamination platforms, Kinoshita and co-workers [38] demonstrated that N -phenylbenzenesulfonamidyl radicals derived from homolysis of a symmetrical sulfonylhydrazide could add to alkenes to give mixtures of products, including sultams. Chemler and co-workers have developed racemic and enantioselective intramolecular Cu(II)-mediated oxidative N -radical cyclizations of alkenyl arylsulfonamides at elevated temperatures (120 °C) to garner benzosultams in good yields [39] , [40] , [41] . Later, Kanai and co-workers [42] reported an intermolecular alkene carboamination reaction of aliphatic alkenes under Cu(I) catalysis and N -fluorobenzenesulfonimide (NFSI) as both a bifunctional reagent, for C–C and C–N bond formation, and an oxidant for the concise synthesis of six-membered sultams. Zhao et al. [43] have disclosed a radical cascade cyclization/allylation of β,γ-unsaturated N -aryl hydrazones that gives dihydropyrazoles and tetrahydropyridazines. Very recently, Zhao et al. [44] have also described a process for a radical 5- exo cyclization/addition/aromatization cascade of β,γ-unsaturated N -tosyl hydrazones under cooperative photocatalysis and cobalt catalysis enabling the synthesis of dihydropyrazole-fused benzosultams. We reasoned that the work outlined above, along with our ongoing interests in alkene carboamination reactions with bifunctional arylsulfonamide reagents [45] , would serve as a basis for developing a catalytic protocol to initiate a carboamination/dearomatization cascade starting from γ,δ-unsaturated N -arylsulfonyl enamides 1 (Fig. 1c ). Ideally, this process would proceed through a transient sulfonamidyl radical intermediate originating from formal removal of the N–H hydrogen atom. This strategy obviates the need for N -pre-functionalization, elevated reaction temperatures, and stoichiometric oxidants. The reaction would lead to the selective synthesis of 1,4-cyclohexadiene-fused sultams. Of note, fused sultams have been shown to exhibit a broad range of biological activities [46] , [47] , [48] . At the outset, we recognized two major challenges in implementing this design strategy. The first was the potential for competitive hydroamination, wherein the vicinal carbon-centered radical that is formed following N -radical cyclization would undergo premature hydrogen atom transfer or reduction to give the hydroamination product [33] , [35] , [36] , [49] , [50] , [51] , [52] , [53] , [54] . The second challenge was rearomatization of the cyclohexadienyl radical intermediate. To circumvent these challenges, it was necessary to identify an efficient photocatalytic system capable of selectively reducing the cyclohexadienyl radical to the cyclohexadienyl anion and reestablish the ground state of the photocatalyst. We believed such challenges could be surmounted with judicious choice of reaction additives and parameters. Herein, we describe the combination of the aforementioned reaction classes, whereby visible light-mediated photoredox catalysis is used to promote and control a sulfonamidyl radical cyclization/dearomatization cascade reaction. 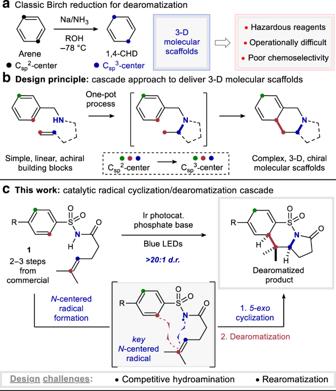Fig. 1: Inspiration and design for our carboamination/dearomatization cascade reaction platform. aThe classic Birch reduction for arene dearomatization.bThe design principle of using a radical cascade approach for arene dearomatization.cThis work: catalytic radical carboamination/dearomatization cascade reactions. Reaction optimization Initially, we chose arylsulfonamide 1a as the model substrate to test the feasibility of the visible light-induced carboamination/dearomatization cascade reaction and representative results are summarized in Table 1 . The expected reaction occured with 1 mol% Ir-photocatalyst A ([Ir(dF(CF 3 ppy) 2 )(5,5′-CF 3 -bpy)]PF 6 , Ir III*/II = 1.68 V versus SCE in MeCN) and 65 mol% of tetrabutylammonium dibutylphosphate base providing the desired 1,4-cyclohexadiene-fused sultam 2a in 48% 19 F-NMR yield and excellent diastereoselectivity (>20:1) following irradiation with blue LEDs in trifluorotoluene (0.2 M) at room temperature (entry 1). 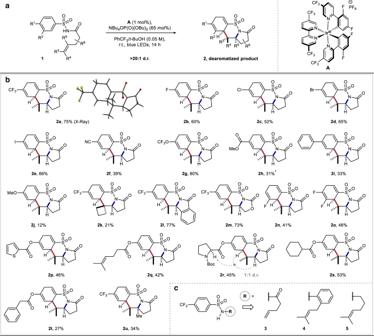Fig. 2: Reaction scope. All yields are isolated yields. Relative configurations of products were assigned by analogy to2a.aGeneral reaction scheme; all reactions were run on 0.2 mmol scale and degassed by sparging with argon for 15 min prior to exposure to optimized conditions.bArylsulfonamide modifications.cControl experiments with differentially substituted alkene side-chains. *Product isolated as an inseparable mixture of diene and arene products (3:1, diene:arene). Dearomatized product 2a was unambiguously characterized by single-crystal X-ray analysis. Other iridium photocatalysts structurally similar to A ( B = [Ir(dF(CF 3 ppy) 2 )(dtbbpy)]PF 6 , Ir III*/II = 1.21 V versus SCE in MeCN; C = [Ir(dF(Meppy) 2 )(dtbbpy)]PF 6 , Ir III*/II = 0.97 V versus SCE in MeCN) [55] , [56] were also effective in these reactions (entries 2, 3), however the reaction yields diminished as the oxidation potential of the excited-state species decreased. Importantly, decreasing the reaction concentration (0.05 M) delivered the desired product in 67% yield (entry 4). Also, the reaction is moderately to equally successful in other solvents (entry 5-7) with tert -butanol providing a noticeable increase in yield (entry 8). A 1:1 mixed solvent system of trifluorotoluene/ tert -butanol (0.05 M) was finally identified as the optimal solvent combination (entry 9). When the reactions were run using conditions developed by Rovis, relying on step-wise deprotonation/oxidation [37] , no product was isolated (See Supplementary Tables 1 and 2 for complete optimization details). Control reactions of 1a lacking photocatalyst, base, or light were uniformly unsuccessful, and the starting material was recovered unchanged (entries 10–12). Table 1 Reaction optimization and control experiments. Full size table Substrate scope With optimized conditions established, we investigated the generality of this carboamination/dearomatization cascade reaction with a series of diversely substituted arylsulfonamides (Fig. 2 ). For example, arenes bearing various electron-withdrawing ( 2a , 2b , 2f – 2i ), electron-neutral ( 2c – 2e ), and electron-donating ( 2j ) groups delivered the desired dearomatized products in moderate to good yields (12–80%) and with excellent diastereoselectivity (>20:1). Unsurprisingly, the latter electron-rich product 2j was prone to rapid oxidative decomposition leading to diminished yields. Dearomatized product 2h was isolated as an inseparable mixture with the aromatized benzosultam product. Next, we investigated modifications to the alkene tether which allowed for the synthesis of an all-carbon spirocycle ( 2k ), fused tetracycle ( 2l ), and cyclic carbamate ( 2m ) in moderate to good yields (21–77%). Interestingly, 3-fluoro and 3,4-difluoro substituted arylsulfonamide substrates generated single dearomatized regioisomers in good yields ( 2n , 2o ) highlighting the regio- and chemoselective nature of the C–C bond forming cyclization step. Furthermore, this methodology proved tolerant of diverse functionality including electron-rich heterocycles ( 2p ), olefins ( 2q ), amino acids ( 2r ), aliphatic carbocycles ( 2s ), and benzyl groups ( 2t ) selectively furnishing the corresponding dearomatized products in good yields. Lastly, a tetrasubstituted olefin substrate ( 1u ) allowed direct access to dearomatized tert -alkylamine [57] product 2u , suggesting the initial 5- exo N -radical cyclization is tolerant to steric encumbrance. Terminal olefin 3 failed to convert to the desired dearomatized product (Fig. 2c ) likely due to the instability of the resultant vicinal primary radical following C–N bond formation. To probe the importance of the carbonyl moiety and to determine whether it is a necessary functionality for the reaction to proceed, we prepared and subjected o -prenyl aniline derivative 4 and alkyl sulfonamide 5 to the optimized reaction conditions and found they were unreactive, returning the starting material. These experiments highlight the potential importance of the carbonyl moiety for this process to occur by lowering the p K a of the substrate (pK a for 1 ≈ 5) [58] . Fig. 2: Reaction scope. All yields are isolated yields. Relative configurations of products were assigned by analogy to 2a . a General reaction scheme; all reactions were run on 0.2 mmol scale and degassed by sparging with argon for 15 min prior to exposure to optimized conditions. b Arylsulfonamide modifications. c Control experiments with differentially substituted alkene side-chains. *Product isolated as an inseparable mixture of diene and arene products (3:1, diene:arene). Full size image Synthetic applications The richly functionalized 1,4-cyclohexadiene-fused sultams accessible with this methodology can be readily diversified, leveraging the functional groups tolerated by the dearomative cyclization (Fig. 3 ). The N -sulfonyl lactam carbonyl is susceptible to nucleophilic addition and subsequent displacement of the sulfonamide leaving group. Thus, 2d is rapidly converted to bicyclic methyl ester 3d at room temperature in excellent yield when treated with excess K 2 CO 3 in methanol. Reaction of 2d with lithium aluminum hydride in THF directly provides the bicyclic alcohol 4d . Of note, 3d and 4d are the products of the formal intermolecular dearomative reaction between a primary sulfonamide N -centered radical and a γ,δ -unsaturated ester or a bis -homoallylic alcohol, respectively. Palladium-catalyzed Suzuki–Miyaura cross-coupling of 2d with N -methylindole-5-boronic acid under unoptimized anhydrous conditions gave a moderate yield of alkenyl indole 5d . Under similar conditions used to prepare 3d , tricyclic sultam 2s containing alkenyl ester functionality converts in good yield to the γ -sulfamoyl enone 3s as a single diastereomer as revelaed by X-ray crystallographic analysis. Due to the resonance stabilizing effects of the enone on the resulting anion, 3s is deprotonated alpha to the sulfonamide by K 2 CO 3 to give a dienolate that is alkylated by benzyl bromide alpha to the carbonyl. Enone 4s is thus isolated following re-conjugation of the remaining alkene with the ketone. N -benzylated products were not observed. Fig. 3: Synthetic modifications of fused-sultam products. All yields are isolated yields. Conditions: a Sat. aq. K 2 CO 3 , MeOH, rt, 15 min. b LiAlH 4 , THF, −78 °C to room temp., 1.5 h. c 1-(methylindol-5-yl)boronic acid, CsF, PPh 3 , Pd(OAc) 2 , THF, reflux, 14 hr. d K 2 CO 3 , MeOH, rt, 15 min. e K 2 CO 3 , benzyl bromide, DMF, rt, 2 h. Full size image Mechanistic investigations To gain insight into the reaction mechanism, we performed Stern–Volmer luminescence quenching studies with the model substrate 1a (Supplementary Figs. 73 – 76 ). It was revealed that there is no luminescence quenching of the photoexcited state of catalyst A when 1a is used alone, suggesting that direct oxidation, followed by deprotonation, of the substrate is unlikely. This conclusion was further supported by cyclic voltammetry analysis (CH 2 Cl 2 containing 0.1 M NBu 4 PF 6 ) indicating that direct oxidation of substrate 1a occurs at potentials >1.6 V (versus SCE) (Supplementary Fig. 77 ). Comparatively, when tetrabutylammonium dibutylphosphate base is used alone in the Stern–Volmer analysis, significant nonlinear photoluminescence quenching of the photoexcited state of catalyst A is observed. This observation aligns with the reports of Knowles [59] , and others [60] , suggesting the formation of a less emissive iridium-phosphate complex which may be the active ground-state catalytic species in solution. Importantly, no additional photoluminescence quenching is observed upon addition of substrate 1a as one would expect for a MS-CPET process. Cyclic voltammetry studies of 1a in the presence of varying concentrations of monobasic dibutylphosphate base revealed that current response increased for increasing concentrations of phosphate base but did not show a shifted, less positive potential for the oxidation of substrate 1a (Supplementary Fig. 77 ). With no evidence for a MS-CPET process, we next investigated whether sequential sulfonamide deprotonation and one-electron oxidation was the operative mechanism for N -centered radical generation. Deprotonation of 1g with sodium hydride followed by salt metathesis gave the sulfonamidyl anion product [NBu 4 ][1g] . When this compound was exposed to the typical reaction conditions in the absence of phosphate, product 2g was not detected and only starting material was observed by NMR analysis of the crude reaction (Fig. 4a ). This result suggests that single-electron oxidation of a sulfonamidyl anion is not the dominant route to the nitrogen-centered radical. Qualitatively, these results together are consistent with a phosphate radical being generated under the reaction conditions and serving as a hydrogen-atom abstracting species and is at least partly responsible for the generation of the nitrogen radical [61] , [62] . HAT between heteroatoms is known to occur rapidly, even in the presence of weaker C–H bonds [63] . Next, a deuterium labeling experiment was conducted to probe the origin of the additional proton on the carbocycle in the products. By performing the reaction in the presence of tert -BuOD, the desired product ( 2a- D ) was produced in 51% yield with complete deuterium incorporation (Fig. 4b ). This result suggests that the tert -BuOH is serving as a reaction-terminating proton source of a 1,4-cyclohexadienyl anion intermediate in accord with previous mechanistic studies of the classic Birch reduction reaction [64] , [65] . Interestingly, the mechanism for sulfonamidyl radical formation presented herein differs from the proposal by Knowles and co-workers [36] . This observed divergence may be due to differences in acidity between the primary benzenesulfonamides used by Knowles and the N -carbonyl benzenesulfonamides used in this study. Fig. 4: Experiment to probe mechanism and proposed catalytic cycle. a Deprotonated substrate is unreactive under reaction conditions. b Deuterium labeling experiment. c Proposed catalytic cycle. Full size image Proposed catalytic cycle A catalytic cycle accounting for these observations, and those made during reaction optimization, is shown in Fig. 4c . We suspect that the Ir-photocatalyst A and phosphate base first form a ground-state iridium-phosphate complex ( i ). Upon excitation, the Ir-photocatalyst can undergo single-electron transfer from the phosphate salt, generating an oxygen-centered radical ( ii ). Abstraction of the most activated H-atom of the substrate ( iii ) generates a transient sulfonamidyl radical intermediate ( iv ). Next, the N -radical can undergo 5- exo cyclization onto the tethered alkene to furnish a new C–N bond and a vicinal carbon-centered radical ( v ). This alkyl radical is poised to undergo cyclization with the appended arene to generate a stabilized cyclohexadienyl radical ( vi ) that can undergo single-electron reduction by the reduced Ir(II) state of the photocatalyst ( E 1/2 [Ir III /Ir II ]= −1.07 V versus Fc + /Fc) [36] . Favorable proton transfer between the cyclohexadienyl anion and tert -BuOH ( tert -butoxide can then return dibutyl phosphoric acid [66] back to the phosphate salt) should deliver the dearomatized product and regenerate both catalysts. In summary, we have reported the discovery and development of a photoredox-mediated N -centered radical strategy to facilitate a carboamination/dearomatization cascade reaction. Simple γ,δ-unsaturated N -arylsulfonyl enamides were converted into complex and stereodefined 1,4-cyclohexadiene-fused sultams in satisfactory yields and excellent diastereoselectivity. This mild and efficient catalytic system demonstrates a broad substrate scope and high functional group tolerance while avoiding premature hydroamination or undesired rearomatization reactivity. Overall, we believe the photochemical strategy outlined here will inspire future synthetic endeavors aimed at employing simple arene building blocks for the rapid synthesis of complex, three-dimensional molecular frameworks in a single operation. 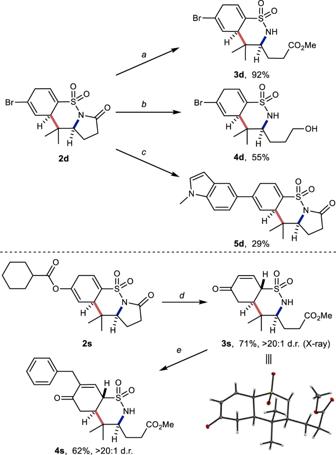Fig. 3: Synthetic modifications of fused-sultam products. All yields are isolated yields. Conditions:aSat. aq. K2CO3, MeOH, rt, 15 min.bLiAlH4, THF, −78 °C to room temp., 1.5 h.c1-(methylindol-5-yl)boronic acid, CsF, PPh3, Pd(OAc)2, THF, reflux, 14 hr.dK2CO3, MeOH, rt, 15 min.eK2CO3, benzyl bromide, DMF, rt, 2 h. 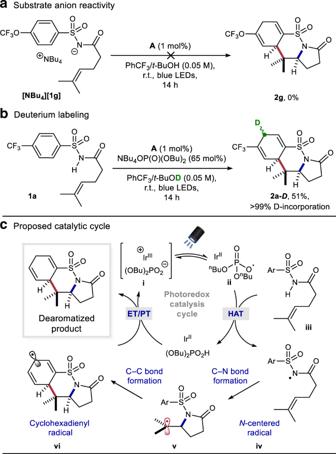Fig. 4: Experiment to probe mechanism and proposed catalytic cycle. aDeprotonated substrate is unreactive under reaction conditions.bDeuterium labeling experiment.cProposed catalytic cycle. Representative procedure To a dry 2-dram vial was added γ,δ-unsaturated N -arylsulfonyl enamide 1 (0.2 mmol), base, (65 mol%), and photocatalyst (1 mol%). The vial contents were then dissolved in a 1:1 mixture of t -BuOH:PhCF 3 (0.05 M). The solution was degassed by sparging with argon for 15 min. The reaction was irradiated with two, H150 blue Kessil lamps positioned ~2 cm away and cooled with an overhead fan for 14 h. The reaction was concentrated in vacuo, loaded onto silica, and purified by flash column chromatography to afford the desired 1,4-cyclohexadiene-fused sultam 2 . No unexpected or unusually high safety hazards were encountered.